Porous organic molecular solids by dynamic covalent scrambling The main strategy for constructing porous solids from discrete organic molecules is crystal engineering, which involves forming regular crystalline arrays. Here, we present a chemical approach for desymmetrizing organic cages by dynamic covalent scrambling reactions. This leads to molecules with a distribution of shapes which cannot pack effectively and, hence, do not crystallize, creating porosity in the amorphous solid. The porous properties can be fine tuned by varying the ratio of reagents in the scrambling reaction, and this allows the preparation of materials with high gas selectivities. The molecular engineering of porous amorphous solids complements crystal engineering strategies and may have advantages in some applications, for example, in the compatibilization of functionalities that do not readily cocrystallize. Most materials with molecular-scale pores are extended networks [1] , [2] , [3] , [4] , [5] , [6] , [7] , [8] , but not solution-processable molecules of the kind commonly prepared by organic chemists. Indeed, the vast majority of organic molecules pack efficiently in the solid state to form structures with minimal void volume. Some organic molecules, however, form void-containing structures such as apohosts or empty beta phases [9] . Calixarenes, in particular, can exhibit 'porosity without pores' [10] , [11] : that is, the solid materials can adsorb guests by cooperative diffusion, despite having isolated voids rather than interconnected pore structures. Permanent, interconnected porosity in discrete organic molecules with low molar mass is rarer [11] and is typically confined to certain ordered molecular crystals [12] , [13] , [14] , [15] , [16] , [17] , [18] , [19] , [20] , [21] , [22] , [23] , [24] . Examples include modified calixarenes [12] , [13] , [14] , 3,3′,4,4′-tetra(trimethylsilylethynyl)biphenyl [15] , tris- o -phenylenedioxycyclotriphosphazene [16] , 4-hydroxyphenyl-2,3-4-trimethylchroman [17] , cucurbit[6]uril [18] , some dipeptides [19] , diyne macrocycles [20] and imine-linked porous organic cages [21] , [22] . Two main strategies have been used to prepare porous organic molecular solids. Macrocycles [12] , [13] , [14] , [18] and molecular cages [21] , [22] possess 'intrinsic' porosity. That is, pores are synthetically prefabricated in the molecules and can be identified by viewing the structure of an isolated molecule. Metal organic polyhedra [25] and heme-like coordination crystals [26] also exhibit intrinsic porosity of this type. Other systems have 'extrinsic' porosity [15] , [16] , [17] , [19] and the pore structure arises purely from the molecular packing. In these cases, porosity may not be obvious from inspection of the isolated molecular structure [24] . Crystal engineering approaches have been used to control the assembly of extrinsically porous molecular solids, for example using directional interactions such as hydrogen bonding [27] , [28] , [29] . A major practical problem for both intrinsically and extrinsically porous molecular crystals is that they often cannot be desolvated while retaining long-range molecular order. More commonly, molecular crystals that contain cavities or channels, such as clathrates and solvates, do not retain their incipient porosity on guest removal and collapse to form a denser phase [11] . This is a key distinction between porous molecular crystals and porous crystalline networks [1] , [2] , [3] , [4] , [5] , [6] , [7] , [8] , where structural collapse may be prevented by extended directional covalent or coordination bonding. An alternative strategy for producing porous materials is to design less symmetrical molecules that do not crystallize and pack inefficiently in the solid state. There has been less focus here in comparison with the preparation of ordered porous solids using crystal engineering [10] , [11] , [12] , [13] , [14] , [15] , [16] , [17] , [18] , [19] , [20] , [21] , [22] , [23] , [24] , [25] , [26] , [27] , [28] , [29] . Polymers of intrinsic microporosity (PIMs), for example, form amorphous microporous solids—that is, amorphous solids with pore dimensions smaller than 2 nm—as a result of their rigid and contorted chain structures [30] , [31] . There are few examples of permanently microporous amorphous solids composed of small organic molecules. One example is the 'paddle-wheel' molecule, Noria, which was shown recently to exhibit porosity in the amorphous state [32] . More recently, microporosity was also invoked for concave molecules with structural similarities to building blocks used to synthesize PIMs [33] . A difference between macromolecules, such as PIMs, and smaller molecules is the increased re-organizational energy barrier, which results from molecular entanglements between polymer chains. As such, permanent porosity in polymers with high free volume may in part be a function of the macromolecular chain structure. For example, the level of porosity in PIM-1 increases with increasing molecular weight [30] . We showed previously that imine-linked cages ( Fig. 1 ) can crystallize to produce organic materials with closed voids (cage 1 ) (ref. 21 ), as well as permanently porous materials with linear channels (cage 2 ) and three-dimensional pore networks (cage 3 ), depending on the cage vertex functionality. Brunauer–Emmett—Teller (BET) surface areas ( SA BET ) as high as 624 m 2 g −1 (cage 3 ) were obtained for these porous molecular crystals. A design principle for enhancing porosity was suggested to us by comparing the crystal structures for cages 1 and 2 . The positionally disordered methyl groups in 2 frustrate molecular packing with respect to unfunctionalized 1 , thus leading to less dense crystal packing in 2 (0.874 versus 1.033 g cm −3 ). This implied that even less symmetrical cages with a combination of functionalized and unfunctionalized vertices might pack even less effectively, thereby enhancing porosity in the solid. A further goal was to produce amorphous molecular materials that do not require special processing conditions such as crystal growth or specific desolvation methodologies [34] to maintain a stable and permanent pore structure. 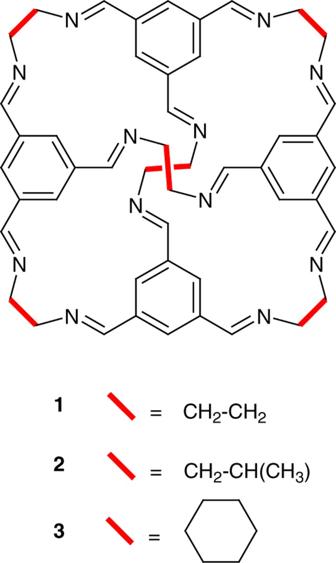Figure 1 Chemical structures of imine-linked cages. Figure 1 Chemical structures of imine-linked cages. Full size image In this study, we present porous organic cages, which are purposefully desymmetrized using dynamic imine–imine interchange reactions to produce a scrambled distribution of molecules that pack together ineffectively. We show that the H 2 /N 2 selectivity can be tuned by varying the composition of this distribution of molecules. Molecular simulations for the amorphous solids suggest that the porosity results from voids running both through and between the cage molecules. Scrambling reactions We exploit here the dynamic nature [35] , [36] of the imine bonds in cages 1 and 3 to form new cage molecules with mixed vertex functionalities. This can be achieved in three different ways. First, mixed cages can be produced directly by [4+6] cycloimination reactions involving more than one vicinal diamine ( Fig. 2a ). For example, the co-reaction of 1,3,5-triformylbenzene (TFB) with a mixture of both 1,2-ethylenediamine (EDA) and (1 R ,2 R )-1,2-cyclohexanediamine (CHDA) leads to an equilibrium distribution of products incorporating both EDA-linked and CHDA-linked vertices in a single cage molecule. These products are designated as 1 n 3 m , where n and m represent the number of EDA and CHDA vertices, respectively. Second, mixed cages may be generated by the reaction of CHDA with the preformed cage, 1 , and this leads to similar distributions of mixed products by vertex exchange reactions. Third, the reaction of cage 1 with cage 3 proceeds slowly in solution at 30 °C to form a comparable 1 n 3 m product distribution by cage–cage interchange reactions. 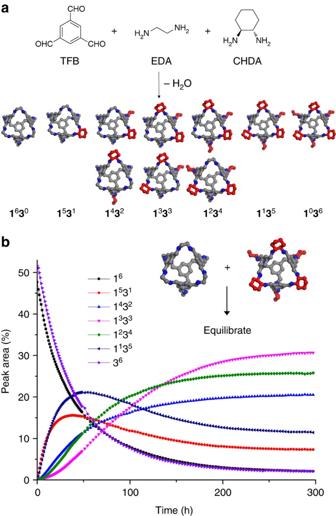Figure 2: Synthesis by direct co-reaction and by dynamic cage–cage scrambling. (a) The direct co-reaction of two different diamines leads to a distribution of molecular shapes; (b) Cage–cage interchange reactions lead to a similar distribution and the kinetics of the scrambling reaction can be followed by high-performance liquid chromatography combined with mass spectrometry and nuclear magnetic resonance spectroscopy. The kinetics of this process is shown in Figure 2b . In general, direct co-reactions and cage–cage interchange reactions have a practical advantage over the amine substitution method, because there is no excess diamine to separate from the resulting product mixture at the end of the reaction. Figure 2: Synthesis by direct co-reaction and by dynamic cage–cage scrambling. ( a ) The direct co-reaction of two different diamines leads to a distribution of molecular shapes; ( b ) Cage–cage interchange reactions lead to a similar distribution and the kinetics of the scrambling reaction can be followed by high-performance liquid chromatography combined with mass spectrometry and nuclear magnetic resonance spectroscopy. 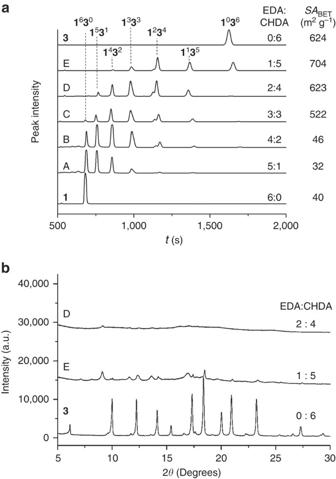Figure 3: Chemical and physical analysis for scrambled cage mixtures. High-performance liquid chromatography (HPLC) analysis (a) and powder X-ray diffraction (PXRD) data (b) for amorphized cage mixtures formed by direct co-reaction of triformylbenzene (TFB) with various ratios of ethylenediamine (EDA) and (1R, 2R)-cyclohexanediamine (CHDA). The Brunauer–Emmett–Teller (BET) surface areas given inawere calculated from nitrogen adsorption isotherms obtained at 77 K. Full size image The co-reaction of TFB with EDA and CHDA was carried out with various EDA:CHDA ratios and the distribution of products was analysed by high-performance liquid chromatography (HPLC) as shown in Figure 3a . The materials were also characterized by nuclear magnetic resonance spectroscopy and mass spectrometry to assign the individual molecular species (see Supplementary Figs S1–S6 ). The equilibrium 1 n 3 m product distribution is controlled by the diamine ratio. High EDA ratios in the reagent mixture lead to a predominance of cage products with high values of n , and vice versa. Three of the products in these distributions have potential to exhibit positional isomerism. The 1 2 3 4 and 1 4 3 2 species could exist as either cis or trans isomers, whereas the 1 3 3 3 species might exist in either meridional ( mer ) or facial ( fac ) forms ( Fig. 2a ). Indeed, chromatographic separation under slightly modified conditions showed two peaks for each of the 1 2 3 4 , 1 3 3 3 and 1 4 3 2 species, suggesting that both of the possible isomeric forms are produced in each case ( Supplementary Fig. S1 ). Figure 3: Chemical and physical analysis for scrambled cage mixtures. High-performance liquid chromatography (HPLC) analysis ( a ) and powder X-ray diffraction (PXRD) data ( b ) for amorphized cage mixtures formed by direct co-reaction of triformylbenzene (TFB) with various ratios of ethylenediamine (EDA) and (1 R , 2 R )-cyclohexanediamine (CHDA). The Brunauer–Emmett–Teller (BET) surface areas given in a were calculated from nitrogen adsorption isotherms obtained at 77 K. Full size image Structural analysis Analysis of the samples by powder X-ray diffraction (PXRD; Fig. 3b ) showed no evidence of long-range molecular order for any of the samples, apart from E which was produced using a 5:1 ratio of CHDA:EDA, in which some crystallization of cage 3 was observed ( Supplementary Fig. S7 ). This was also supported by scanning electron microscopy analysis ( Supplementary Figs S14–S15 ), in which a mixture of crystallites and amorphous particles was observed for E . Gas sorption analysis Samples C – E produced with a ratio of CHDA:EDA ≥3 showed type I gas sorption isotherms [37] and demonstrated substantial permanent surface areas as measured by nitrogen sorption at 77 K ( SA BET =522–704 m 2 g −1 ). The porosity in these samples is predominantly microporous with between 75 and 80% of the total pore volume being accounted for by pores with diameters smaller than 2 nm ( Supplementary Figs S16–S17 , Supplementary Table S2 ). The highest surface area (sample E ; 704 m 2 g −1 ) exceeds that measured for crystalline cage 3 (624 m 2 g −1 ) (ref. 21 ). Likewise, a sample produced by the dynamic equilibration of the preformed cages 1 and 3 was completely amorphous and showed a surface area of 818 m 2 g −1 ( Fig. 4a ). These surface areas are comparable with linear PIMs [30] , [31] , [33] , although unlike PIMs these cage materials are not macromolecules. The amorphous cage materials also adsorb a number of different gases other than N 2 (see Supplementary Table S3 ). For example, samples A – E , adsorb amounts of CO 2 in the range 1.60–1.93 mmol g −1 (7.0–8.7 wt%) at 298 K and 1 bar. 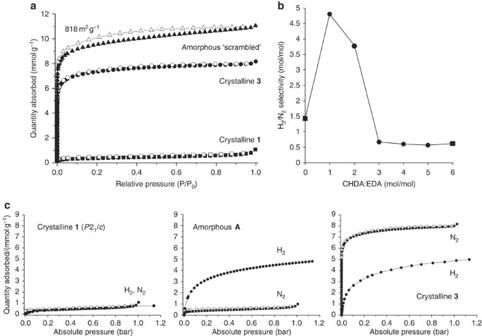Figure 4: Cage scrambling allows enhanced porosity and tunable gas selectivity. (a) Nitrogen adsorption isotherms (filled symbols) and desorption isotherms (open symbols) for crystalline cages1and3and an amorphous sample,F, which was prepared by a cage–cage interchange reaction between1and3(Fig. 2b). This demonstrates that cage 'scrambling' leads to enhanced porosity (SABET=818 m2g−1). Gas selectivity data (b) for amorphous cage mixtures prepared by co-reaction compared with single-component crystalline analogues. SampleA(CHDA:EDA=1:5) exhibits the highest H2selectivity over N2. The relevant sorption isotherms (c) show how H2sorption (circle symbols), but not N2sorption (square symbols), is switched 'on' in amorphousAwith respect to crystalline1. Figure 4: Cage scrambling allows enhanced porosity and tunable gas selectivity. ( a ) Nitrogen adsorption isotherms (filled symbols) and desorption isotherms (open symbols) for crystalline cages 1 and 3 and an amorphous sample, F , which was prepared by a cage–cage interchange reaction between 1 and 3 ( Fig. 2b ). This demonstrates that cage 'scrambling' leads to enhanced porosity ( SA BET =818 m 2 g −1 ). Gas selectivity data ( b ) for amorphous cage mixtures prepared by co-reaction compared with single-component crystalline analogues. Sample A (CHDA:EDA=1:5) exhibits the highest H 2 selectivity over N 2 . The relevant sorption isotherms ( c ) show how H 2 sorption (circle symbols), but not N 2 sorption (square symbols), is switched 'on' in amorphous A with respect to crystalline 1 . Full size image Physical stability The porosity in the materials is robust: for example, all samples were heated to 120 °C for 15 h to outgas them before gas sorption analysis. The amorphous materials also have reasonable thermal stability with decomposition onset temperatures of around 350 °C as measured by thermogravimetric analysis, equivalent to their crystalline analogues [21] ( Supplementary Fig. S24 ). Crucially, for A – D there is no evidence for crystallization of individual components over time, nor does the porosity appear to be sensitive to processing conditions such as the rate at which the solvent is removed. Control experiments for sample D also showed that the nature of the porosity is not strongly sensitive to the solvent used in the synthesis or isolation of the material ( Supplementary Figs S25–S26 ). Tuneable guest selectivity Unlike porous molecular crystals [12] , [13] , [14] , [15] , [16] , [17] , [18] , [19] , [20] , [21] , [22] , [23] , [24] , [25] , [26] , these amorphous solids comprise a distribution of molecular species, which can be controlled by the diamine feed ratio ( Fig. 3a ). It is therefore possible to use synthesis to tune the gas sorption properties by varying this molecular distribution. For example, the gas selectivity is a strong function of the EDA:CHDA ratio ( Fig. 4b ). Materials with low CHDA ratios ( A , B ) adsorb much more H 2 than N 2 at cryogenic temperatures. Sample A in particular (EDA:CHDA=1:5) adsorbs around five times as much H 2 as N 2 , mole per mole, as measured at 1 bar. As shown in Figure 4c , sample A has a much better H 2 selectivity than either of the crystalline solids 1 ( 1 6 3 0 ) and 3 ( 1 0 3 6 ). Atomistic simulations We rationalize the enhanced gas sorption properties of these amorphous materials both in terms of the inherent, prefabricated pores in the cage molecules, and the ineffective packing that results from the distribution of molecular shapes. This was explored by constructing an atomistic model for sample D ( Fig. 5a,b ). A periodic simulation cell was built containing 32 cage molecules chosen to represent the numerical distribution of species observed by HPLC. The simulated bulk density for the model was 0.766 g cm −3 , which is close to that measured for the sample experimentally (0.716 g cm −3 ) using a combination of gas sorption and helium pyknometry [6] . Interconnected pore channels can be identified in the model, which permeate the simulation cell, running both through and between the cages. This suggests a combination of intrinsic and extrinsic porosity in contrast to analogous crystalline cage materials in which the porosity runs either exclusively between (cage 2 ) or through (cage 3 ) the permanent cage cavities [21] . A solvent accessible surface area [38] of 577 m 2 g −1 was calculated for this model, which is commensurate with the experimental surface area, SA BET , for D of 623 m 2 g −1 . Although it is difficult to probe experimentally for these amorphous solids, the contribution of inter-cage pore volume with respect to internal cage volume can be estimated from this atomistic model. In the model for sample D ( Fig. 5a,b ), 80% of the total free volume in the simulation cell arises from voids between the badly packed cages, compared with 20% calculated for the internal cage volume itself. By contrast, calculations for crystalline 3 based on X-ray crystal structures show that 37.6% of the pore volume can be attributed to voids between cages and 63.4% to the internal cage voids ( Supplementary Fig. S27 ). As such, we suggest that the porosity in D results predominantly from this large increase in inter-cage void volume in the amorphous solid, which more than compensates for the fact that some internal cage volume is probably 'lost' as a result of broken connectivity between the cage voids ( Supplementary Fig. S28 ). 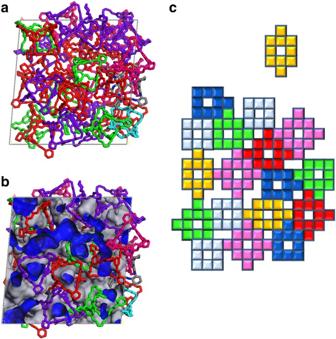Figure 5: Inefficient packing enhances porosity. (a) Atomistic simulation for amorphous sampleD(EDA:CHDA=2:4). An amorphous cell was constructed containing 33 cage molecules (1×1531, 5×1432, 9×1333, 12×1234, 5×1135, 1×1036) chosen to represent the molecular distribution as calculated from HPLC peak areas (Fig. 3a). The Connolly surface (b) is also shown using a probe radius of 1.82 Å. Analysis suggests that around 80% of the void volume is generated by cavities between the cages, rather than the internal cage volume itself. (c) The frustrated packing in this system has analogies with computer games such as Tetris, which are based on the problem of tiling space with a set of two-dimensional shapes. Figure 5: Inefficient packing enhances porosity. ( a ) Atomistic simulation for amorphous sample D (EDA:CHDA=2:4). An amorphous cell was constructed containing 33 cage molecules (1× 1 5 3 1 , 5× 1 4 3 2 , 9× 1 3 3 3 , 12× 1 2 3 4 , 5× 1 1 3 5 , 1× 1 0 3 6 ) chosen to represent the molecular distribution as calculated from HPLC peak areas ( Fig. 3a ). The Connolly surface ( b ) is also shown using a probe radius of 1.82 Å. Analysis suggests that around 80% of the void volume is generated by cavities between the cages, rather than the internal cage volume itself. ( c ) The frustrated packing in this system has analogies with computer games such as Tetris, which are based on the problem of tiling space with a set of two-dimensional shapes. Full size image The poor packing of the scrambled cage mixture is shown schematically in Figure 5c . Based on this 'Tetris model', we speculate that desymmetrized cage analogues with more bulky vertex substituents might exhibit even higher levels of porosity than those observed here. As it stands, these molecules are the most porous non-polymeric amorphous solids produced to date. Although the surface areas do not match highly porous networks, the synthetic control over gas selectivity rivals that obtained in crystalline materials. The scope for rational design in such amorphous solids differs from, say, isoreticular MOFs [2] in which physical properties are correlated directly with a repeating long-range ordered structure. Nevertheless, structure property relationships can be learned, if not at this stage actually designed: for example, average micropore size in samples A – E can be tuned as a function of EDA:CHDA ratio, and this translates into tunable (albeit not ab initio predictable) gas selectivity behaviour. More advanced methods for computational structure prediction might allow us in the future to carry out the in silico design of molecular libraries which pack to give specific, tailored pore size distributions. The molecular solubility of these desymmetrized cages gives rise to processing advantages. For example, preliminary results show that the molecular pores can be imbibed into various porous supports, such as cellulose filter paper, to introduce a degree of microporosity into otherwise macroporous materials. Our results also suggest the possibility of modular 'mix and match' strategies in which a number of different molecular pores are combined in a single-amorphous solid, each perhaps containing a different chemical functionality [39] , without satisfying the stringent requirements of co-crystallization [40] . Materials 1,3,5-Triformylbenzene was purchased from Manchester Organics. All other chemicals were purchased from Sigma-Aldrich and used as received, unless otherwise stated. Direct co-reactions Dichloromethane (DCM; 25 ml) was slowly added to TFB (100 mg, 0.62 mmol) in a sample vial at room temperature. Under these conditions, the TFB did not dissolve immediately. A solution of EDA in DCM (5 ml) and a solution of CHDA in DCM (5 ml) were added (amounts listed in Supplementary Table S1 ). After 5 days, a clear homogeneous solution was observed with no undissolved material being present. The product was obtained by solvent evaporation. The crude product was filtered washed with ethylacetate to remove any unreacted starting materials. The product was air dried overnight before analysis. Typical yield after washing 55–60%. Cage–cage interchange reaction between 1 and 3 Cage 3 (100 mg, 0.0895 mmol) was dissolved in chloroform (10 ml). Cage 1 (100 mg, 0.1262 mmol) was also dissolved in a separate volume of chloroform (10 ml). The reaction was carried out in an HPLC autosampler for ease of sampling and the two solutions were kept separate until the start of the HPLC analysis. The solutions were mixed immediately before analysis in a proportion, which achieved a 1:1 molar ratio of 1 : 3 (10 ml of the cage 3 solution + 7.1 ml of the cage 1 solution). HPLC chromatograms were then measured every hour for the first 48 h and subsequently every 3 h up to a total reaction time of 300 h. The reaction was maintained at a constant temperature of 30 °C. The procedure for isolation of the product was the same as that described above for co-reactions. Reaction of 1 with CHDA Cage 1 (50 mg, 0.0631 mmol) was dissolved in 5 ml of chloroform. CHDA (54 mg, 0.473 mmol) was dissolved in 5 ml of chloroform (molar ratio of CHDA:cage 1 =7.5:1). The cage 1 solution was added directly to the CHDA solution at room temperature. Simulations A model for amorphous sample D was constructed using Materials Studio 5.0 (Accelrys). The model was built in three stages. First, cage molecules were constructed for each cage isomer combination using the crystallographic structure of cage 1 as a template (obtained from the Cambridge Crystallographic Database with reference numbers CCDC 707056) [21] . For cage 1 itself ( 1 6 3 0 ), the structure was assumed to be tetrahedral, as per the crystalline structure CCDC 707056, although we cannot preclude the presence of non-tetrahedral conformers in the amorphous solid [41] . Next, an amorphous cell was constructed containing 33 of the cage molecules (1× 1 5 3 1 , 5× 1 4 3 2 , 9× 1 3 3 3 , 12× 1 2 3 4 , 5× 1 1 3 5 , 1× 1 0 3 6 ) chosen to represent the molecular distribution as calculated from HPLC peak areas ( Fig. 3a ). The trans isomer of the 1 4 3 2 molecule, the cis isomer of 1 2 3 4 molecule and the mer isomer of the 1 3 3 3 molecule chosen arbitrarily for this simulation. The structures of these 32 cage molecules were fixed as rigid bodies and the amorphous cell was loaded to a density of 0.3 g cm −3 using the Universal Forcefield (UFF) [42] . The model was then geometry optimized under an external pressure using the Forcite module and COMPASS force field [43] . The external pressure was continually ramped up until the simulation density was higher than a 'target' bulk density. The target bulk density, ρ app was obtained from the equation W 0 =1/ ρ app −1/ ρ tr , where W 0 is the micropore volume (0.22 cm 3 g −1 ; pore volume <2 nm) and ρ tr is the absolute density, measured by helium pycnometry (0.844 g cm −3 ) [6] , [44] , [45] . Finally, the model was allowed to fully relax in the absence of an external pressure and the simulation density (0.767 g cm −3 ) remained relatively close to the 'target' density (0.712 g cm −3 ). This atomistic simulation gives an indication of the likely cage packing mode in the amorphous sample, D , although there are a number of limitations, which prevent more quantitative predictions. For example, any gas sorption arising from sample morphology at higher relative pressures, or from pores that may be present which are larger than the simulation cell, is not catered for in this simulation. Nuclear magnetic resonance Solution 1 H nuclear magnetic resonance (NMR) spectra were recorded at 400.13 MHz using a Bruker Avance 400 NMR spectrometer (Bruker). 13 C NMR spectra were recorded at 100.6 MHz. Thermogravimetric analysis Thermogravimetric analysis was carried out using a Q5000IR analyzer (TA instruments) with an automated vertical overhead thermobalance. The samples were heated at the rate of 5 °C min −1 . Scanning electron microscopy High resolution imaging of the crystal morphology was achieved using a Hitachi S-4800 cold Field Emission Scanning Electron Microscope (Hitachi). The dry samples were prepared on 15 mm Hitachi M4 aluminium stubs using either silver dag or an adhesive high purity carbon tab. The samples were then coated with a 2 nm layer of gold using an Emitech K550X automated sputter coater. The field emission scanning electron microscope measurement scale bar was calibrated against certified standards. Imaging was conducted at a working distance of 8 mm and a working voltage of 3 kV using a mix of upper and lower secondary electron detectors. Powder X-ray diffraction PXRD data were collected on a PANalytical X'pert pro multi-purpose diffractometer in transmission Debye–Scherrer geometry operating with a Cu anode at 40 kV 40 mA. Samples were ground and mounted as loose powder onto a transparent film and spun at 2 s per rotation. PXRD patterns were collected in two 1-h scans with a step size of 0.013° 2 θ and scan time of 115 s per step over 5–50° 2 θ . The incident X-ray beam was conditioned with 0.04 rad Soller slits and an antiscatter slit of 1/2°. The diffracted beam passed through an automatic antiscatter slit (5 mm), 0.04 rad Soller slits and Ni filter before processing by the PIXcel detector operating in scanning mode. Gas sorption analysis All samples were tested with gases of the following purities: hydrogen (99.9995%—BOC gases), carbon dioxide (SCF grade—BOC gases) and methane (ultrahigh purity—BOC). Surface areas and pore size distributions were measured by nitrogen adsorption and desorption at 77.3 K using a Micromeritics ASAP 2020 volumetric adsorption analyzer (Micromeritics). Samples were degassed at offline at 120 °C for 15 h under vacuum (10 −5 bar) before analysis, followed by degassing on the analysis port under vacuum, also at 80 °C. Carbon dioxide isotherms were measured at 273 and 293 K using a Micromeritics 2020 volumetric adsorption analyzer (Micromeritics) using the same degassing procedure. Mass spectrometry Samples were analysed by matrix-assisted laser desorption/ionization time-of-flight spectrometry. A 10:1 ratio of matrix/sample was dissolved in DCM (10 mg ml −1 ) and this was drop coated onto the microtitre plate before analysis. The matrix used was trans -2-[3-(4- tert -butylphenyl)-2-methyl-2-propenylidene]malononitrile. The instrument used was an AXIMA Confidence—MALDI MS (Shimadzu Biotech) fitted with a 50 Hz N 2 laser. Thermo Scientific Accela U-HPLC system Columns used for the analysis of co-reaction samples and inter-cage exchange reactions between 1 and 3 were Hypersil GOLD Phenyl, 150×4.6 mm, 5 μm (SN 0591330K, Lot 9193) linked to Hypersil GOLD, 150×4.6 mm, 5 μm, (SN 1284371N, Lot 9231). The mobile phase was ethanediol/MeOH, 5/95 (premixed) at a flow rate was 0.5 ml min −1 . The injection volume was 10 μl and the sample concentration was 0.1 mg ml −1 in MeOH. The column oven temperature was set to 30 °C. Analytical columns used for resolution of isomer peaks ( Supplementary Fig. S1 ) were Waters XBridge phenyl 4.6×150 mm, 5 μm (Waters) and XBridge C18 4.6×100 mm, 5 μm. The mobile phase used 80–95% MeOH in 0.1% NH 4 OH. Detection for HPLC analysis was conducted at 236 nm. How to cite this article: Jiang, S. et al . Porous organic molecular solids by dynamic covalent scrambling. Nat. Commun. 2:207 doi: 10.1038/ncomms1207 (2011).